Jumonji demethylases moderate precocious flowering at elevated temperature via regulation ofFLCinArabidopsis As sessile organisms, plants have evolved multiple mechanisms to respond to environmental changes to improve survival. Arabidopsis plants show accelerated flowering at increased temperatures. Here we show that Jumonji-C domain-containing protein JMJ30 directly binds to the flowering-repressor FLOWERING LOCUS C ( FLC ) locus and removes the repressive histone modification H3 lysine 27 trimethylation (H3K27me3). At elevated temperatures, the JMJ30 RNA and protein are stabilized, and FLC expression is maintained at high levels to prevent extreme precocious flowering. The double mutant of JMJ30 and its homologue JMJ32 , grown at elevated temperatures, exhibits an early-flowering phenotype similar to the flc mutant, which is associated with increased H3K27me3 levels at the FLC locus and decreased FLC expression. Furthermore, ectopic expression of JMJ30 causes an FLC -dependent late-flowering phenotype. Taken together, JMJ30/JMJ32-mediated histone demethylation at the FLC locus constitutes a balancing mechanism in flowering control at warm temperatures to prevent premature early flowering. Unlike animals, plants are sessile organisms that stay in the same location throughout their life cycle and are continually exposed to fluctuating ambient conditions, thus highlighting the importance of rapid adaptation to increase the odds of survival. Plants have evolved a myriad of mechanisms to perceive environmental conditions and respond to these changes, as deviations from normal growth conditions could stress the plants and have severe effects on their growth and development. The inevitable changes to the global climate represent an emerging threat, as many plants are highly sensitive to temperature fluctuations [1] . A slight increase or decrease in ambient temperature could affect the growth rate, organ maturation and function, and flowering transition [2] , [3] . Under normal growth conditions, upon reaching a certain developmental stage and perceiving the right environmental cues, plants would undergo a floral transition. In Arabidopsis , this switch from a vegetative to a reproductive phase is controlled by four pathways, and all inputs congregate on a few key floral regulators: the floral repressor FLOWERING LOCUS C ( FLC ), which acts upstream and represses the downstream floral inducers FLOWERING LOCUS T ( FT ) and SUPPRESSOR OF OVEREXPRESSION OF CONSTANS 1 ( SOC1 ) [4] , [5] , [6] , [7] . In addition, recent findings have revealed a few players involved in a fifth flowering pathway that is responsive to ambient temperature changes and has been called the thermosensory pathway. Elevated ambient temperatures accelerate flowering by reducing the repressive H2A.Z nucleosome occupancy at the FT locus, which then allows the transcription factor PHYTOCHROME INTERACTING FACTOR 4 (PIF4) to bind and activate FT [8] , [9] . On the other hand, the MADS-box heterocomplex containing SHORT VEGETATIVE PHASE (SVP) and a temperature-dependent isoform of FLOWERING LOCUS M (FLM) represses flowering at lower temperatures [10] , [11] , [12] , [13] , [14] . The floral repressor FLC was also shown to delay flowering during short exposures to non-freezing cold temperatures [15] . These findings suggest the interplay of multiple thermosensory mechanisms in controlling flowering in response to ambient temperature fluctuations. Considering how the important ‘decision’ of the vegetative-reproductive phase change centres on just a few genes, it is not surprising that in addition to regulation by transcription factors, many chromatin remodelling mechanisms have evolved to tightly control the expression of these genes. Accelerated flowering by vernalization treatment involves the epigenetic silencing of FLC through the Polycomb Group (PcG)-mediated gradual deposition of the trimethylation of lysine 27 of histone H3 (H3K27me3) [16] . Even when plants are grown under normal non-vernalized conditions, the PRC2-like complex containing CURLY LEAF, EMBRYONIC FLOWER 2 and FERTILIZATION-INDEPENDENT ENDOSPERM represses FLC expression during vegetative development [17] . In addition to H3K27me3, FLC expression is also regulated by repressive H3K9me2 marks, activating H3K4me3/H3K36me3 marks, and histone acetylation [5] , [18] , [19] . These crosstalks of histone marks at the locus depend on the interplay between histone methyltransferases and histone demethylases [20] , [21] . There are two known classes of histone demethylases, and only the Jumonji-C (JmjC) domain-containing proteins have the ability to demethylate trimethylated histones. There are 21 JUMONJI ( JMJ ) genes in Arabidopsis , which can be categorized into five groups, namely the KDM5/JARID1, KDM4/JHDM3/JMJD2, KDM3/JHDM2, JMJD6 and JmjC domain-only group, based on their JmjC domain sequences and domain architectures [22] , [23] . Members from the same group show similar target specificity for histone modifications [24] , [25] , [26] , [27] , [28] , [29] , [30] , [31] , [32] . One of the histone modifications, the repressive PcG-mediated H3K27me3, plays a key role in gene repression and developmental regulation, and is actively and dynamically deposited and removed in plants [33] . However, although the demethylases for H3K27me3, UTX and JMJD3 were found years ago in animals [34] , there is no Arabidopsis homologue in the same KDM6/JMJD3 group. Only recently, members from the KDM4/JHDM3/JMJD2 group, RELATIVE OF EARLY FLOWERING 6 (REF6) in Arabidopsis and JMJ705 in rice, were reported as H3K27me3 demethylases [29] , [35] . Early flowering at high temperatures mediated by the thermosensory pathways is considered to be an adaptive trait to maximize the reproductive success. However, flowering too early without sufficient vegetative growth may risk not having enough nutrients and resources to support seed maturation. Here we show that JMJ30/AT3G20810 and JMJ32/AT3G45880, two members of the JmjC domain-only group of JMJ proteins, function as H3K27 demethylases and regulate FLC expression in Arabidopsis . Our results suggest that JMJ30/JMJ32-mediated FLC regulation may constitute a balancing mechanism that controls flowering time to ensure reproductive success at elevated temperatures. FLC prevents precocious flowering at elevated temperatures The flowering time of the flc-3 null mutant is indistinguishable from Columbia wild-type (WT) plants when grown at 22 °C under long day (LD, 16-h light/8-h dark) conditions ( Fig. 1a,b ) [36] , [37] . However, when grown at 29 °C LD conditions, flc-3 plants flowered earlier than WT plants with the leaf number ratio (29 °C/22 °C) of 0.51 for flc-3 and 0.69 for WT ( Fig. 1a,b ), suggesting that FLC contributes to preventing precocious flowering at elevated temperatures [38] . Although FLC expression is low in WT plants that lack a functional FRIGIDA ( FRI ) [38] , expression analyses are still able to detect basal FLC expression, which gradually decreases during vegetative development ( Fig. 1c ) [27] . To determine whether FLC temporal expression level is affected by elevated temperatures, we analysed FLC expression in plants grown at 22 °C and 29 °C under LD conditions at 5, 9 and 13 days-after-germination (DAG) before the plants undergo the bolting process. We observed that after shifting to 29 °C at 3 DAG, FLC expression was initially comparable between plants grown at 22 °C and 29 °C at 5 DAG ( Fig. 1c ). FLC expression decreases gradually at 9 and 13 DAG in plants grown under both the 22 °C and 29 °C conditions, but this FLC downregulation is significantly attenuated in plants grown at 29 °C ( Fig. 1c ). This result showed that FLC repression during vegetative development is delayed during growth at elevated temperatures. 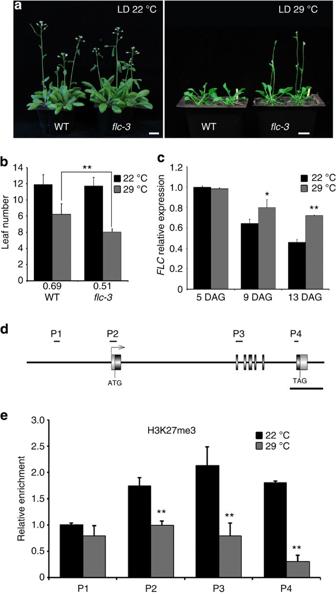Figure 1:FLCis a suppressor of thermal induction of flowering. (a)flc-3flowers at a similar time as WT when grown in LD 22 °C, but flowering is accelerated inflc-3when grown under LD 29 °C conditions. Representative 30-day-old plants (LD 22 °C) or 23-day-old plants (LD 29 °C) are shown for comparison. Scale bar, 1 cm. (b) Total primary rosette leaves before bolting in WT andflc-3plants grown under LD 22 °C and 29 °C conditions were counted (two independent experiments with 15–20 plants each). Numbers below graph indicate leaf number ratio (29 °C/22 °C). Bars indicate standard deviation (s.d.); two-tailed Student’st-test, **P<0.01. (c)FLCmRNA levels in 5, 9 and 13 DAG seedlings grown under LD 22 °C and 29 °C conditions. Relative fold changes to 5 DAG seedlings grown under 22 °C conditions are presented. Bars indicate s.d. of three biological replicates; two-tailed Student’st-test, *P<0.05, **P<0.01. (d) Schematic drawing of theFLCgenome structure showing regions amplified by primers used for ChIP analysis. Scale bar, 1 kb. (e) ChIP analysis of H3K27me3 enrichment at theFLClocus in 8 DAG WT seedlings grown under LD 22 °C and 29 °C conditions. An anti-H3 antibody was used as a control. Bar indicates standard error of the mean (s.e.m.) of three biological replicates; two-tailed Student’st-test, **P<0.01. Figure 1: FLC is a suppressor of thermal induction of flowering. ( a ) flc-3 flowers at a similar time as WT when grown in LD 22 °C, but flowering is accelerated in flc-3 when grown under LD 29 °C conditions. Representative 30-day-old plants (LD 22 °C) or 23-day-old plants (LD 29 °C) are shown for comparison. Scale bar, 1 cm. ( b ) Total primary rosette leaves before bolting in WT and flc-3 plants grown under LD 22 °C and 29 °C conditions were counted (two independent experiments with 15–20 plants each). Numbers below graph indicate leaf number ratio (29 °C/22 °C). Bars indicate standard deviation (s.d. ); two-tailed Student’s t -test, ** P <0.01. ( c ) FLC mRNA levels in 5, 9 and 13 DAG seedlings grown under LD 22 °C and 29 °C conditions. Relative fold changes to 5 DAG seedlings grown under 22 °C conditions are presented. Bars indicate s.d. of three biological replicates; two-tailed Student’s t -test, * P <0.05, ** P <0.01. ( d ) Schematic drawing of the FLC genome structure showing regions amplified by primers used for ChIP analysis. Scale bar, 1 kb. ( e ) ChIP analysis of H3K27me3 enrichment at the FLC locus in 8 DAG WT seedlings grown under LD 22 °C and 29 °C conditions. An anti-H3 antibody was used as a control. Bar indicates standard error of the mean (s.e.m.) of three biological replicates; two-tailed Student’s t -test, ** P <0.01. Full size image We wondered whether this delayed repression is regulated at the chromatin level. As FLC reduction during the developmental switch from vegetative to reproductive phase is known to be regulated by the repressive H3K27me3 (refs 16 , 17 ), we performed chromatin immunoprecipitation (ChIP) assays to assess the level of H3K27me3 at the FLC locus at 8 DAG, which is on the brink of floral transition occurring at 9 DAG [39] ( Fig. 1d,e ). Compared with WT plants grown under 22 °C LD conditions, WT plants grown at 29 °C showed reduced H3K27me3 enrichment at the FLC locus ( Fig. 1e ). This finding indicates that delayed FLC repression at elevated temperatures is associated with the reduction of the repressive H3K27me3 at the FLC locus. Taken together, these results suggest that H3K27me3-associated histone modifiers may participate in the thermosensory pathway by regulating FLC expression at elevated temperatures to control flowering in moderation. Mutation of jmj30 and jmj32 promotes flowering at 29 °C The lower levels of H3K27me3 at the FLC locus at elevated temperatures and the increased level of FLC expression led us to conjecture that the effect may be maintained through the action of H3K27me3 demethylases. However, FLC expression is upregulated rather than downregulated in the loss-of-function mutant of the only known Arabidopsis H3K27me3 demethylase, REF6 (refs 29 , 40 ). Hence, we reasoned that there might be other JMJ proteins that may remove the H3K27me3 repressive marks at the FLC locus. Among the five groups of Arabidopsis JMJ proteins, four of them (KDM5/JARID1, KDM4/JHDM3/JMJD2, KDM3/JHDM2 and JMJD6) have been implicated as histone demethylases specific for other histone modifications, such as H3K4 and H3K9 (refs 22 , 23 , 24 , 25 , 26 , 27 , 28 , 29 , 30 , 31 , 32 ). Little is known about the enzymatic function of the JmjC domain-only group that contains no other known functional protein domains but the catalytic JmjC domain, except their role in circadian regulation [41] , [42] . To elucidate the function of this group, we used two previously described loss-of-function mutants for JMJ30 : jmj30-1 (SAIL_811_H12) and jmj30-2 (GK-454C10) [41] , [42] , and isolated one T-DNA insertional mutant for JMJ32 : jmj32-1 (SALK_003313; Fig. 2a ). No full-length JMJ30 mRNA was detected for either allele, and we decided to use jmj30-2 for subsequent experiments, as it produced no partial fragments ( Fig. 2b , Supplementary Fig. 1a,b ). No full-length JMJ32 mRNA was detected in jmj32-1 , but partial fragments were still detectable ( Fig. 2b , Supplementary Fig. 1a,c ). However, because the T-DNA is inserted at the catalytic JmjC domain in jmj32-1 ( Fig. 2a ), it likely produces a null mutant. Under the standard growth conditions (22 °C LD), neither the single nor the double jmj30-2 jmj32-1 (herein jmj30 jmj32 ) mutants differed from WT in terms of flowering time, which is similar to the flc mutant’s lack of a phenotype under standard growth conditions ( Figs 1a,b and 2c,d ). However, we found that the jmj30 jmj32 double mutant flowered earlier than the WT when grown under elevated temperatures with the decreased leaf number ratio (29 °C/22 °C) of 0.52 compared with 0.69 in WT, but no obvious difference in phyllochron length ( Fig. 2c,d ), as was observed in flc ( Fig. 1a,b ). We then studied the response of jmj30 jmj32 to elevated temperature in short days (SDs, 8-h light/16-h dark) and observed the enhanced early-flowering phenotype compared with WT grown under the same conditions, with the leaf number ratio (29 °C/22 °C) of 0.19 for jmj30 jmj32 and 0.24 for WT ( Supplementary Fig. 2a,b ). 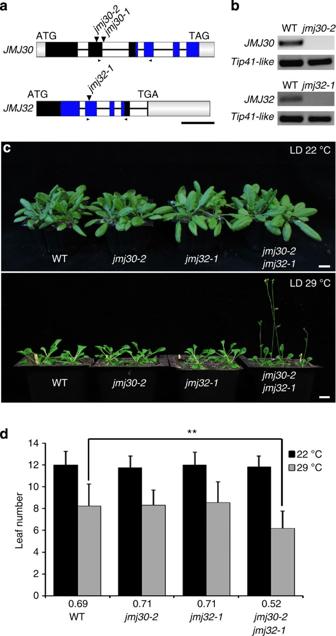Figure 2:jmj30 jmj32loss-of-function mutant accelerates flowering at elevated temperatures. (a) Schematic drawings ofJMJ30andJMJ32genomic structures. Grey boxes indicate the 5′and 3′ untranslated region (UTR). Black boxes indicate exons, whereas blue boxes indicate exons coding for the JmjC domain. White boxes with a line indicate introns. T-DNA insertion sites are marked by downward pointing arrowheads above the schematic diagrams, whereas smaller arrowheads show primers used for RT–PCR. Scale bar, 500 bp. (b) RT–PCR ofJMJ30andJMJ32in WT,jmj30-2andjmj32-1.Tip-41 likeis shown as an internal control. (c)jmj30-2,jmj32-1andjmj30-2 jmj32-1flower at a similar time as WT when grown under LD 22 °C conditions, butjmj30-2 jmj32-1showed accelerated flowering when grown under LD 29 °C conditions. Representative 25-day-old plants (LD 22 °C) or 23-day-old plants (LD 29 °C) were shown as comparison. Scale bar, 1 cm. (d) Total primary rosette leaves before bolting in WT,jmj30-2,jmj32-1andjmj30-2 jmj32-1plants grown under LD 22 °C and 29 °C conditions were counted (two independent experiments with 15–20 plants each). Numbers below graph indicate leaf number ratio (29 °C/22 °C). Bars indicate s.d.; two-tailed Student’st-test, **P<0.01. Figure 2: jmj30 jmj32 loss-of-function mutant accelerates flowering at elevated temperatures. ( a ) Schematic drawings of JMJ30 and JMJ32 genomic structures. Grey boxes indicate the 5′and 3′ untranslated region (UTR). Black boxes indicate exons, whereas blue boxes indicate exons coding for the JmjC domain. White boxes with a line indicate introns. T-DNA insertion sites are marked by downward pointing arrowheads above the schematic diagrams, whereas smaller arrowheads show primers used for RT–PCR. Scale bar, 500 bp. ( b ) RT–PCR of JMJ30 and JMJ32 in WT, jmj30-2 and jmj32-1 . Tip-41 like is shown as an internal control. ( c ) jmj30-2 , jmj32-1 and jmj30-2 jmj32-1 flower at a similar time as WT when grown under LD 22 °C conditions, but jmj30-2 jmj32-1 showed accelerated flowering when grown under LD 29 °C conditions. Representative 25-day-old plants (LD 22 °C) or 23-day-old plants (LD 29 °C) were shown as comparison. Scale bar, 1 cm. ( d ) Total primary rosette leaves before bolting in WT, jmj30-2 , jmj32-1 and jmj30-2 jmj32-1 plants grown under LD 22 °C and 29 °C conditions were counted (two independent experiments with 15–20 plants each). Numbers below graph indicate leaf number ratio (29 °C/22 °C). Bars indicate s.d. ; two-tailed Student’s t -test, ** P <0.01. Full size image We next proceed to look at the expression profile of the flowering time genes. We collected 5, 9 and 13 DAG seedling samples grown at 29 °C LD conditions at the end of the light photoperiod. The jmj30 jmj32 double mutant decreased FLC expression at all tested time points ( Fig. 3a ). Furthermore, the trend of decreased FLC expression at 13 DAG is similar in jmj30 jmj32 seedlings grown at 29 °C ( Fig. 3a ) and WT grown at 22 °C ( Fig. 1c ). The other thermosensory mediator SVP was not significantly affected ( Fig. 3b ). In contrast, the expression of the florigen FT and another floral promoter SOC1 were increased especially in 13 DAG seedlings of jmj30 jmj32 relative to WT at 29 °C LD ( Fig. 3c,d ). These results align with reports that the FLC-SVP complex represses FT in leaves and SOC1 in both leaves and shoot apical meristems [43] . AGAMOUS-LIKE 24 ( AGL24 ) and CONSTANS ( CO ) were not significantly affected in jmj30 jmj32 ( Fig. 3e,f ). In short, the results suggest that jmj30 jmj32 mutations decrease FLC expression at elevated temperatures, and this effect appears to upregulate the floral integrators FT and SOC1 , which are two common targets of FLC. 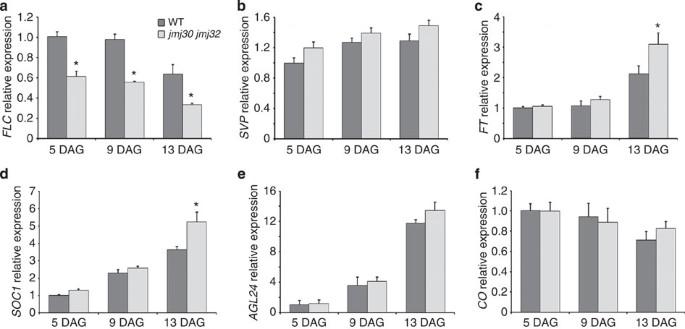Figure 3: Expression profiles of flowering time genes. (a–f) RT–qPCR-based expression profiles of (a)FLC, (b)SVP, (c)FT, (d)SOC1, (e)AGL24and (f)COin 5, 9 and 13 DAG seedlings of WT andjmj30-2 jmj32-1grown under LD 29 °C conditions. Relative fold changes to WT 5 DAG seedlings are presented. Bars indicate s.d. of three biological replicates; two-tailed Student’st-test, *P<0.05. Figure 3: Expression profiles of flowering time genes. ( a – f ) RT–qPCR-based expression profiles of ( a ) FLC , ( b ) SVP , ( c ) FT , ( d ) SOC1 , ( e ) AGL24 and ( f ) CO in 5, 9 and 13 DAG seedlings of WT and jmj30-2 jmj32-1 grown under LD 29 °C conditions. Relative fold changes to WT 5 DAG seedlings are presented. Bars indicate s.d. of three biological replicates; two-tailed Student’s t -test, * P <0.05. Full size image Characterization of JMJ30 and JMJ32 To further reveal the function of JMJ30 and JMJ32, we characterized their spatial expression patterns. Transcript profiling data deposited at the Arabidopsis eFP Browser suggest that JMJ30 and JMJ32 are rather ubiquitously expressed at the rosette leaves, shoot apex and developing flowers ( Supplementary Fig. 3a,b ) [44] . To confirm this, we extracted RNA from different tissues of WT plants, and by reverse transcription–PCR (RT–PCR), we concluded that JMJ30 and JMJ32 were expressed in all tested tissue types, namely, seedlings, roots, rosette leaves, cauline leaves, stems and inflorescences ( Supplementary Fig. 4a ) [22] . JMJ30 was highly expressed in leaves, whereas JMJ32 expression showed no appreciable difference across the various tissue types. Next, to better understand the spatial distribution of JMJ30 and JMJ32 at the protein level, constructs harbouring their upstream promoter and downstream sequences plus the genomic coding sequence (6.1-kb JMJ30 and 5.3-kb JMJ32) fused with the β-glucuronidase (GUS) reporter gene were transformed into WT plants ( Fig. 4a ). This genomic fragment of JMJ30, when fused with the short haemagglutinin (HA) epitope tag, was sufficient to rescue the jmj30 jmj32 early-flowering phenotype at 29 °C LD ( Supplementary Fig. 5a,b ), indicating that the fragment contains all the cis -elements necessary to capture the endogenous expression pattern. Histochemical GUS staining results showed that JMJ proteins were rather ubiquitously expressed, including in the leaves, roots and inflorescences ( Fig. 4b,c ). Furthermore, JMJ30 and JMJ32 expression in the vasculature of leaves overlapped with the expression patterns of their putative targets FLC [45] , FT [46] and SOC1 (refs 47 , 48 ), and FLC is known to directly repress FT and SOC1 in the leaf veins [43] . 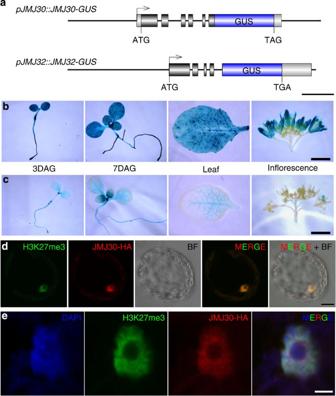Figure 4: Spatial expression patterns of JMJ30 and JMJ32. (a) Schematic drawings ofpJMJ30::JMJ30-GUSandpJMJ32::JMJ32-GUS. Exons are represented by black boxes, and GUS is represented by blue boxes. Lines indicate promoter, introns and 3′ downstream regions. Scale bar, 1 kb. (b,c) Histochemical GUS staining of (b)pJMJ30::JMJ30-GUSand (c)pJMJ32::JMJ32-GUStransgenic lines. 3 and 7 DAG seedlings, rosette leaves and inflorescences were stained overnight. Scale bars, 2 mm. (d,e) Immunolocalization of H3K27me3 and JMJ30-HA in protoplasts generated fromjmj30-2 pJMJ30::JMJ30-HAtransgenic lines. (d) JMJ30-HA localization resembles that of H3K27me3 in the nucleus. Scale bar, 10 μm. (e) Image shows enlarged view of a nucleus. Scale bar, 2.5 μm. Figure 4: Spatial expression patterns of JMJ30 and JMJ32. ( a ) Schematic drawings of pJMJ30::JMJ30-GUS and pJMJ32::JMJ32-GUS . Exons are represented by black boxes, and GUS is represented by blue boxes. Lines indicate promoter, introns and 3′ downstream regions. Scale bar, 1 kb. ( b , c ) Histochemical GUS staining of ( b ) pJMJ30::JMJ30-GUS and ( c ) pJMJ32::JMJ32-GUS transgenic lines. 3 and 7 DAG seedlings, rosette leaves and inflorescences were stained overnight. Scale bars, 2 mm. ( d , e ) Immunolocalization of H3K27me3 and JMJ30-HA in protoplasts generated from jmj30-2 pJMJ30::JMJ30-HA transgenic lines. ( d ) JMJ30-HA localization resembles that of H3K27me3 in the nucleus. Scale bar, 10 μm. ( e ) Image shows enlarged view of a nucleus. Scale bar, 2.5 μm. Full size image To study the sub-cellular localization of JMJ30 and JMJ32, we transiently overexpressed JMJ-VENUS in tobacco Nicotiana benthamiana . We observed that JMJ30 and JMJ32 localized not only to the nucleus but also occasionally to the endoplasmic reticulum and cytoplasm ( Supplementary Fig. 4b ) as reported previously [41] , which could be artefacts from the overexpression of the JMJ proteins. We thus generated an endogenous pJMJ30 promoter-driven JMJ30-HA in jmj30-2 , which complements the early-flowering phenotype of jmj30 jmj32 ( Supplementary Fig. 5a,b ), and performed an immunolocalization assay using anti-HA and anti-H3K27me3 antibodies on its protoplasts. We observed that JMJ30-HA localized primarily to the nucleus, consistent with its role as a histone demethylase, and its expression pattern resembled that of H3K27me3 ( Fig. 4d,e ). Moreover, immunolocalization assay performed using the extracted nuclei from jmj30-2 pJMJ30::JMJ30-HA showed that JMJ30-HA localization to the euchromatin but not to the 4',6-diamidino-2-phenylindole (DAPI)-dense heterochromatic chromocentres, resembling reported localization of H3K27me3 (refs 49 , 50 ), and this localization was not affected by the ambient temperature ( Supplementary Fig. 4c ). JMJ30 and JMJ32 specifically demethylate H3K27me2/3 Proteins that have the catalytic JmjC domain are known to be histone demethylases [51] , and JMJ30-HA localization that resembled the euchromatic histone marks inspired us to study the biochemical function of these histone demethylases. We first determined whether they could demethylate methylated histones in vitro . We transiently overexpressed 35S::JMJ30-HA in tobacco leaves and immunoaffinity-purified the protein using anti-HA agarose beads. Using these purified proteins, an in vitro demethylase assay was carried out. We incubated calf thymus histones with JMJ30-HA proteins, together with reported JmjC cofactors Fe(II) ions and α-ketoglutarate (α-KG). Indeed, western blotting analyses indicated that JMJ30-HA was able to demethylate oligonucleosomes at H3K27me3 and H3K27me2 but not at H3K27me1 ( Fig. 5a ). 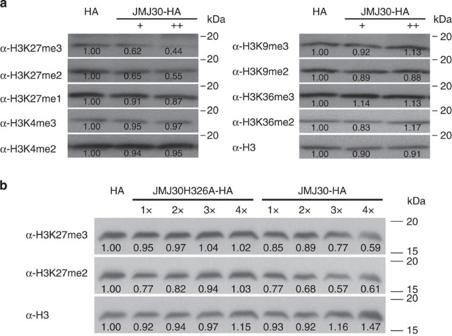Figure 5: JMJ30 demethylates H3K27me2/3in vitro. (a) Immunoaffinity-purified JMJ30-HA was co-incubated with substrate calf thymus histone and cofactors Fe(II) ions and α-KG at 37 °C for 4 h. Immunoblot analysis of histone demethylase activity of JMJ30 was performed using antibodies indicated to the left. The anti-H3 antibody is used as loading control. (b) A mutated version of JMJ30-HA (JMJ30H326A-HA) was unable to demethylate H3K27me2/3in vitrowhen a conserved Fe(II)-binding histidine residue in the JmjC domain was replaced by alanine. Numbers indicate relative band intensity compared with control reaction (HA) performed using an anti-HA precipitate from WT. At least two biological replicates were performed and one set of the data is shown here. Figure 5: JMJ30 demethylates H3K27me2/3 in vitro . ( a ) Immunoaffinity-purified JMJ30-HA was co-incubated with substrate calf thymus histone and cofactors Fe(II) ions and α-KG at 37 °C for 4 h. Immunoblot analysis of histone demethylase activity of JMJ30 was performed using antibodies indicated to the left. The anti-H3 antibody is used as loading control. ( b ) A mutated version of JMJ30-HA (JMJ30H326A-HA) was unable to demethylate H3K27me2/3 in vitro when a conserved Fe(II)-binding histidine residue in the JmjC domain was replaced by alanine. Numbers indicate relative band intensity compared with control reaction (HA) performed using an anti-HA precipitate from WT. At least two biological replicates were performed and one set of the data is shown here. Full size image To investigate the demethylase activity of JMJ30 further, we purified a mutated version of JMJ30-HA (JMJ30H326A-HA), in which one of its conserved Fe(II)-binding histidine residues in the JmjC domain was mutated to alanine. We found that the effect of JMJ30H326A-HA on H3K27me2/3 was completely abolished by the mutation ( Fig. 5b ). To address their substrate specificity, we looked at their ability to demethylate other histone methylation marks. Consistent with the previously reported group-specific characteristics of JMJ proteins, we did not see noticeable demethylation activity for H3K4me2/3, H3K9me2/3 and H3K36me2/3 in the in vitro demethylase assay ( Fig. 5a ). The results indicate that JMJ30 can specifically demethylate H3K27me2/3 in vitro and that its activity is dependent on its JmjC domain. Next, to confirm whether JMJ30 and JMJ32 can exert this demethylase activity in plants, we transiently overexpressed 35S::JMJ30-HA and 35S::JMJ32-HA , and their respective mutated versions of 35S::JMJ30H326A-HA and 35S::JMJ32H174A-HA in Arabidopsis leaf protoplasts. Immunostaining assays were then conducted on the isolated nuclei using anti-H3K27me3 and anti-HA antibodies to observe their demethylase activity in vivo . We found that the overexpression of JMJ30-HA reduced H3K27me3 levels, however, overexpression of the mutated JMJ30H326A-HA has no effect on H3K27me3 methylation ( Supplementary Fig. 6a,b ). Similarly, the H3K27me3 levels were reduced in nuclei overexpressing JMJ32-HA but not in the mutated JMJ32H174A-HA-expressing nuclei ( Supplementary Fig. 6c,d ). Taken together, these results indicate that JMJ30 and JMJ32 function as H3K27me3 demethylases. JMJ30 overexpression delays flowering by upregulating FLC To further elucidate the function of JMJ30, we overexpressed JMJ30-HA in WT plants and confirmed that 35S::JMJ30-HA transgenic lines exhibit constitutive overexpression of JMJ30 and late-flowering phenotypes at 22 °C LD conditions ( Supplementary Fig. 7a–d ) [41] . To understand the effects of JMJ30 overexpression at a molecular level, we checked the expression profiles of the flowering time genes in two independent transgenic lines grown at 22 °C under inductive LD conditions. Supporting the phenotypic observations, the floral repressor FLC is strongly increased in the 35S::JMJ30-HA overexpression lines ( Fig. 6a ). We also found that FT and SOC1 are mildly downregulated ( Fig. 6a ). As FLC is the common repressor of the two floral integrators [43] and was most significantly affected, the increase in FLC expression is likely to be the main reason for the late-flowering phenotype. 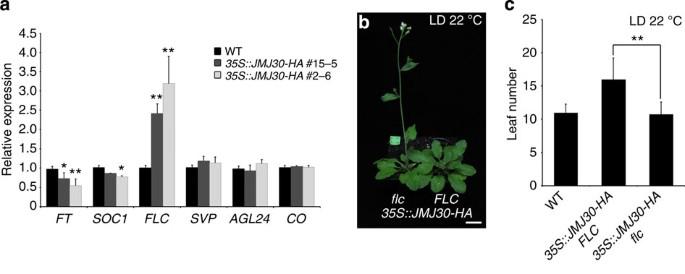Figure 6: Overexpression of JMJ30 leads to delayed flowering. (a) mRNA expression levels of flowering time genes in WT and two independent lines of35S::JMJ30-HA. Relative fold changes to WT are presented. Bars indicate s.d. of three biological replicates; two-tailed Student’st-test, *P<0.05, **P<0.01. (b) Introduction offlcmutation rescues the late-flowering phenotype of35S::JMJ30-HA. Scale bar, 1 cm. (c) Total primary rosette leaves before bolting in WT,35S::JMJ30-HAand35S::JMJ30-HA flcplants grown under LD 22 °C conditions were counted (two independent experiments with 20–50 plants each). Bars indicate s.d.; two-tailed Student’st-test, **P<0.01. Figure 6: Overexpression of JMJ30 leads to delayed flowering. ( a ) mRNA expression levels of flowering time genes in WT and two independent lines of 35S::JMJ30-HA . Relative fold changes to WT are presented. Bars indicate s.d. of three biological replicates; two-tailed Student’s t -test, * P <0.05, ** P <0.01. ( b ) Introduction of flc mutation rescues the late-flowering phenotype of 35S::JMJ30-HA . Scale bar, 1 cm. ( c ) Total primary rosette leaves before bolting in WT, 35S::JMJ30-HA and 35S::JMJ30-HA flc plants grown under LD 22 °C conditions were counted (two independent experiments with 20–50 plants each). Bars indicate s.d. ; two-tailed Student’s t -test, ** P <0.01. Full size image Based on the results, we hypothesized that FLC is a target of JMJ30. To test whether FLC is genetically necessary for JMJ30 functions, we performed a genetic analysis by crossing 35S::JMJ30-HA with flc-3 . Introduction of the flc mutation largely abolished the late-flowering phenotype of 35S::JMJ30-HA , and 35S::JMJ30-HA flc-3 flowered at a similar time as flc-3 or WT plants ( Fig. 6b,c ). Taken together, these results support the notion that JMJ30 and FLC function in the same genetic pathway that regulates flowering time and that FLC functions downstream of the histone demethylase JMJ30. JMJ30 and JMJ32 regulate H3K27me3 at the FLC locus Our results suggested that JMJ30 functions as an H3K27me2/3 demethylase in vitro ( Fig. 5a,b ) and in vivo ( Supplementary Fig. 6a,b ), and that FLC may be a direct target of JMJ30 ( Figs 3a and 6a–c ). We were interested in verifying whether the increased FLC expression in JMJ30 overexpression lines is similarly reflected in the H3K27 methylation status of the FLC locus. ChIP assays were carried out comparing the H3K27me3 levels between WT and our 35S::JMJ30-HA plants, and we found that the repressive H3K27me3 levels were decreased at the FLC locus in the 35S::JMJ30-HA lines ( Fig. 7a ), which is consistent with the increased FLC expression levels ( Fig. 6a ). 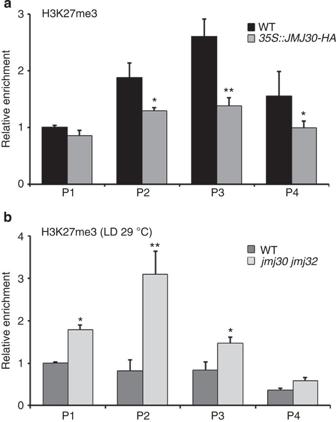Figure 7: The repressive H3K27me3 on theFLClocus is affected by JMJ30 and JMJ32. (a,b) ChIP analysis of H3K27me3 enrichment on theFLClocus in (a) 8 DAG WT and35S::JMJ30-HAseedlings grown under LD 22 °C conditions and (b) 8 DAG WT andjmj30 jmj32seedlings grown under LD 29 °C conditions. An anti-H3 antibody was used as a control. Bar indicates s.e.m. of three biological replicates; two-tailed Student’st-test, *P<0.05, **P<0.01. Figure 7: The repressive H3K27me3 on the FLC locus is affected by JMJ30 and JMJ32. ( a , b ) ChIP analysis of H3K27me3 enrichment on the FLC locus in ( a ) 8 DAG WT and 35S::JMJ30-HA seedlings grown under LD 22 °C conditions and ( b ) 8 DAG WT and jmj30 jmj32 seedlings grown under LD 29 °C conditions. An anti-H3 antibody was used as a control. Bar indicates s.e.m. of three biological replicates; two-tailed Student’s t -test, * P <0.05, ** P <0.01. Full size image We next measured H3K27me3 enrichment at the FLC locus in jmj30 jmj32 and WT grown under 29 °C LD conditions, in which the jmj30 jmj32 double mutant showed decreased FLC expression and accelerated flowering ( Figs 2c,d and 3a ). Consistent with its expression, we found that the H3K27me3 levels at the FLC locus are increased in jmj30 jmj32 at 29 °C ( Fig. 7b ). Taken together, these results indicate that JMJ30 and JMJ32 demethylate H3K27me3 at the FLC locus to activate FLC expression at elevated temperatures. Prolonged JMJ30 activity directly regulates FLC expression The ability of JMJ30 to affect the H3K27me3 level on FLC chromatin leads us to speculate that JMJ30 may directly bind to the FLC locus and demethylate the repressive mark. ChIP assays were conducted using the overexpression 35S::JMJ30-HA transgenic line and the endogenous promoter-driven pJMJ30::JMJ30-HA jmj30-2 line grown at 29 °C under LD conditions. We immunoprecipitated the epitope-tagged JMJ30-HA protein using anti-HA agarose to assess the level of JMJ30-HA binding across the FLC chromatin region. Compared with WT plants, we found that JMJ30-HA associates with FLC chromatin directly in both lines, with the P2 region near the transcriptional start site showing the highest levels of binding enrichment ( Fig. 8a ; Supplementary Fig. 8 ). 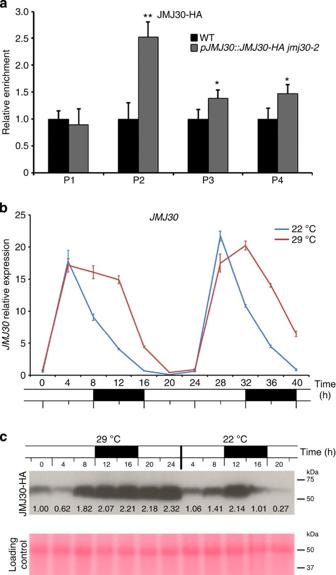Figure 8: Prolonged JMJ30 activity under elevated temperature directly regulatesFLCexpression. (a) ChIP analysis of JMJ30-HA enrichment at theFLClocus in 8 DAG WT andjmj30-2 pJMJ30::JMJ30-HAseedlings. JMJ30-HA directly binds near the transcriptional start site of theFLClocus. A mouse IgG was used as control. Bar indicates s.e.m. of three biological replicates; two-tailed Student’st-test, *P<0.05, **P<0.01. (b)JMJ30mRNA levels in WT seedlings grown under LD 22 °C and 29 °C conditions, measured over 40 h (h). Relative fold changes to 0 h are presented. Bars indicate s.d. of three biological replicates. (c) Relative JMJ30-HA protein levels over 24 h examined by western blot using anti-HA-HRP antibody. Total proteins fromjmj30-2 pJMJ30::JMJ30-HAseedlings grown under LD 22 °C and 29 °C conditions were used. Ponceau Red-stained membrane is shown as a loading control. Numbers indicate relative band intensity compared with 29 °C 0 h sample. Two biological replicates were performed and one set of the data is shown here. Figure 8: Prolonged JMJ30 activity under elevated temperature directly regulates FLC expression. ( a ) ChIP analysis of JMJ30-HA enrichment at the FLC locus in 8 DAG WT and jmj30-2 pJMJ30::JMJ30-HA seedlings. JMJ30-HA directly binds near the transcriptional start site of the FLC locus. A mouse IgG was used as control. Bar indicates s.e.m. of three biological replicates; two-tailed Student’s t -test, * P <0.05, ** P <0.01. ( b ) JMJ30 mRNA levels in WT seedlings grown under LD 22 °C and 29 °C conditions, measured over 40 h (h). Relative fold changes to 0 h are presented. Bars indicate s.d. of three biological replicates. ( c ) Relative JMJ30-HA protein levels over 24 h examined by western blot using anti-HA-HRP antibody. Total proteins from jmj30-2 pJMJ30::JMJ30-HA seedlings grown under LD 22 °C and 29 °C conditions were used. Ponceau Red-stained membrane is shown as a loading control. Numbers indicate relative band intensity compared with 29 °C 0 h sample. Two biological replicates were performed and one set of the data is shown here. Full size image To further elucidate the mechanism underlying the positive regulation of FLC expression at elevated temperatures by JMJ30, we were interested in JMJ30 mRNA and protein expression and stability at 22 °C and 29 °C. JMJ30 mRNA diurnal expression has been previously reported [41] , [42] . Taking samples from WT seedlings grown at 22 °C and 29 °C under LD condition every 4 h, we found that JMJ30 expression peaked approximately 4 h before dark for both conditions, and the peak levels in the JMJ30 diurnal expression were not significantly affected by the temperature. However, we found that the width of the peak broadened under the 29 °C conditions ( Fig. 8b ), which could be due to prolonged expression or increased mRNA stability. To test if the protein expression of JMJ30 is similarly affected, we did a western blot with total proteins extracted from jmj30-2 pJMJ30::JMJ30-HA using an anti-HA-HRP antibody. Under standard growth conditions (22 °C LD), the peak of the JMJ30-HA protein accumulation at the beginning of dark was slightly delayed compared with its mRNA expression, and JMJ30-HA was degraded quickly after that ( Fig. 8c ). At 29 °C, not only was the JMJ30-HA protein accumulation lengthened, it was also more stable as it persisted much longer than expected based on mRNA expression ( Fig. 8b,c ). To confirm this, we performed a protein stability assay by pre-treating the seedlings with cycloheximide to prevent de novo protein synthesis, and adding the proteasome inhibitor MG132 at the end of the light photoperiod. We collected the samples at different time points and found that the rapid degradation of JMJ30-HA at 22 °C was inhibited by the addition of the proteasome inhibitor MG132 ( Supplementary Fig. 9 ), suggesting that the proteasome-dependent JMJ30-HA degradation is impaired at higher temperatures. These results suggested that the strongly prolonged JMJ30 expression at elevated temperatures may allow JMJ30 to bind and demethylate H3K27me3 at the FLC locus, thus maintaining a transcriptionally permissive chromatin status. JMJ30-regulated genes are enriched for H3K27me3 targets To investigate whether JMJ30 overexpression and jmj30 jmj32 loss-of-function mutants influence gene transcription at a global level, we performed expression profiling using NimbleGen 12 × 135K arrays. Compared with WT, 469 genes were downregulated and 657 genes were upregulated in jmj30 jmj32 under 29 °C LD conditions ( Supplementary Data 1 , NCBI Gene Expression Omnibus GSE51898). On the other hand, 516 genes were upregulated and 588 genes were downregulated in 35S::JMJ30-HA compared with WT ( Supplementary Data 2 ). The transcriptome analyses suggested that despite only showing flowering phenotypes, the loss-of-function and overexpression of JMJ30 did affect global expression profiles. Previous studies identified that at least 25% (27.70% of genes analysed in our microarray) of the Arabidopsis genome is targeted by H3K27me3 (refs 33 , 52 ), and our study showed that JMJ30 and JMJ32 are H3K27me3 demethylases. We found that 193 of the 469 (41.15%) total downregulated genes in jmj30 jmj32 and 213 of the 516 (41.28%) genes upregulated in 35S::JMJ30-HA overlapped with reported H3K27me3-regulated genes ( Fig. 9a , Supplementary Data 1 and 2 ) [33] , [52] . Moreover, the genes downregulated in jmj30 jmj32 showed enrichment for PcG targets (41.15%, Fisher’s exact test, P -value=3.499 × 10 −10 ) compared with the upregulated genes (201 out of 657, 30.59%, Fisher’s exact test, P -value=0.0565). Gene ontology analysis of the H3K27me3 targets affected by JMJ30/JMJ32 (shaded in Fig. 9a ) revealed that, in terms of molecular function, genes involved in transcription factor activity (Fisher’s exact test, P -value=8.899 × 10 −3 ) were more enriched, and there were slight enrichment in transcription, DNA-dependent genes in terms of biological process (Fisher’s exact test, P -value=6.074 × 10 −2 ; Fig. 9b ). The 40% correlation between reported H3K27me3 targets and our transcriptome profiling suggested that JMJ30/JMJ32-mediated gene regulation positively influences gene expression by demethylating the repressive H3K27me3, thereby contributing to gene de-repression. 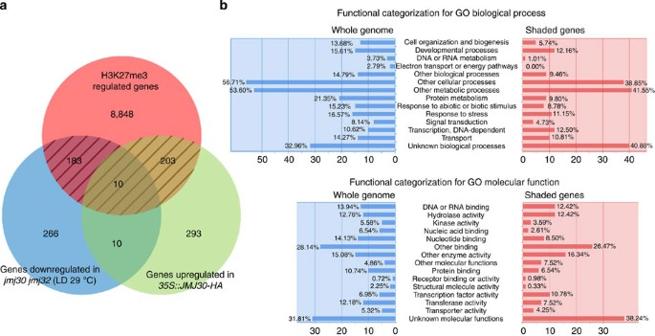Figure 9: Hundreds of genes are regulated byJMJ30/JMJ32. (a) Diagram showing overlap of genes downregulated injmj30 jmj32grown under LD 29 °C conditions, genes upregulated in35S::JMJ30-HAand reported H3K27me3-regulated genes33,52. Genes showing a 1.5-fold change within a 90% confidence interval were considered to be differentially expressed. (b) Functional categorization for Gene Ontology of genes shaded ina. Figure 9: Hundreds of genes are regulated by JMJ30/JMJ32 . ( a ) Diagram showing overlap of genes downregulated in jmj30 jmj32 grown under LD 29 °C conditions, genes upregulated in 35S::JMJ30-HA and reported H3K27me3-regulated genes [33] , [52] . Genes showing a 1.5-fold change within a 90% confidence interval were considered to be differentially expressed. ( b ) Functional categorization for Gene Ontology of genes shaded in a . Full size image In this study, we revealed that the histone modifiers JMJ30 and JMJ32 demethylate H3K27me3 marks at the FLC locus to delay the repression of the floral repressor at elevated temperatures. In the flowering pathways, FLC is the central repressor that represses two floral integrators, FT and SOC1 , in Arabidopsis [43] . We showed that JMJ30 specifically demethylates H3K27me2/3 in vitro ( Fig. 5a,b ) and in vivo ( Supplementary Fig. 6 ). Moreover, jmj30 jmj32 double mutant showed accelerated flowering when grown under 29 °C LD or SD conditions ( Fig. 2c,d , Supplementary Fig. 2a,b ), a temperature below the one used in basal thermo-tolerance experiments [53] . On the other hand, overexpression of JMJ30-HA led to an obvious late-flowering phenotype ( Supplementary Fig. 7a–d ). The mutation of fri flc leads to early-flowering under LD ( Fig. 1a,b ) or SD [38] conditions with increased temperatures. Accordingly, in both jmj30 jmj32 and 35S::JMJ30-HA lines, we noticed that FLC expression was the most obviously affected ( Figs 3a and 6a ). The direct binding of JMJ30-HA to the transcriptional start site of the FLC locus shows that FLC is a direct target of JMJ30 ( Fig. 8a ; Supplementary Fig. 8 ). Moreover, the genetic rescue of the late-flowering phenotype of JMJ30 overexpression by introducing the flc mutation strengthens the notion that JMJ30 functions through FLC to help regulate flowering time ( Fig. 6b,c ). Our work shows the importance of the balancing act between PcG-mediated histone methylation and JMJ30/JMJ32-mediated histone demethylation on H3K27 in controlling the expression of genes such as FLC . Under the functional FRI background, FRI jmj30 jmj32 showed only a modest decrease of FLC at 3-weeks-after-germination at 29 °C LD ( Supplementary Fig. 10 ). A strong transcription activity driven by activators such as FRI may negatively affect the deposition of the repressive H3K27me3 marks at the FLC locus as previously suggested [54] , possibly masking the effect of JMJ30/JMJ32. FRI -activated FLC is gradually silenced through vernalization with the accumulation of H3K27me3 (ref. 16 ). It would hence be interesting to study the effect of JMJ30/32 on vernalization under the FRI background. JMJ30 transcript shows diurnal circadian rhythm ( Fig. 8b ) [41] , [42] . JMJ30/JMJ32-dependent FLC delayed repression at elevated temperatures led us to examine whether the higher activity of JMJ30 is mediated through increased expression levels or a shift in circadian rhythms. We found that JMJ30 diurnal expression is increased by maintaining the high peak before dropping to start another cycle ( Fig. 8b ) and the protein is further stabilized ( Fig. 8c ; Supplementary Fig. 9 ). Although FLC itself is not controlled by circadian regulation, we reasoned that the increased accumulation of the JMJ30 protein at a higher temperature can help maintain the FLC locus in a transcriptionally permissive state. Our data showed that instability of JMJ30 protein at 22 °C is mediated by proteasomal degradation pathway, which is blocked by the proteasome inhibitor MG132 or when the plants are grown at 29 °C ( Supplementary Fig. 9 ). Our future work includes the search for interacting partners of JMJ30 in its temperature-dependent behaviour. Expression profiling showed that 396 out of thousands of H3K27me3-regulated genes are upregulated in 35S::JMJ30-HA and/or downregulated in jmj30 jmj32 . The fact that the expression profiles of many H3K27me3-regulated genes are not affected, suggests that JMJ30 and JMJ32 may only target a subset of H3K27me3-regulated genes. Because JMJ30 and JMJ32 contain only the catalytic JmjC domain, the activity of these histone modifiers may be dependent on the availability of a recruiter to the target genes. Furthermore, this JmjC domain-only group contains another member, JMJ31/AT5G19840, which has a different variant for one of its key α-KG-binding amino acids and is thus likely to be enzymatically inactive [51] . Hence, the biological function of JMJ31 remains to be elucidated. In animals, the H3K27me3 demethylases are developmentally essential, and loss-of-function mutants of the demethylases usually lead to severe developmental defects and lethality. In mouse, JMJD3 inactivation results in perinatal lethality because of respiratory failure [55] , whereas the loss of the zebrafish Utx1 leads to posterior developmental defects [56] . In Caenorhabditis elegans , the utx-1 loss-of-function mutant leads to sterility and embryonic lethality [57] , whereas loss of the JMJD3 homologue causes abnormal gonad development [34] . In Arabidopsis , one member of the KDM4/JHDM3/JMJD2 group, REF6 , has been shown to target the floral inducer FT [29] . Because FT functions downstream of FLC , ref6-1 is supposed to be epistatic to jmj30-2 jmj32-1 , as was observed in the late-flowering phenotype of ref6-1 jmj30-2 jmj32-1 ( Supplementary Fig. 11 ). It is of note that the ref6-1 jmj30-2 jmj32-1 triple mutant showed no severe developmental defects other than its late-flowering phenotype ( Supplementary Fig. 11 ). The lack of phenotype suggests that other H3K27me3 demethylases exist in addition to these JMJ proteins, that the feedback loop to the histone methylation is robust and flexible, or that the developmental plasticity is greater in plants than in animals. JMJ30 and JMJ32 differ from REF6 both in their JmjC domain sequences and their lack of the JmjN domain [22] . Moreover, the JmjC domains of JMJ30, JMJ32 and REF6 showed considerable diversifications even among members of the same group, except for the highly conserved amino acids close to the Fe(II) and α-KG-binding residues [22] . Such variations within the catalytic domains of JMJ proteins have been reported in human JHDM1 and JMJD2A, both of which carry out H3K36me2 demethylation [58] . Thus, it is not uncommon for JMJ proteins with diverse variation within the JmjC domain to target the same substrate, as in the case of REF6, JMJ30 and JMJ32 in Arabidopsis . Crystal structures of JMJ30, JMJ32, REF6 and their cognate substrate (H3K27me3) may be helpful to verify substrate specificity-determining residues. In addition to the floral integrators, FT and SOC1 , FLC also binds and regulates many stress-responsive genes, such as the cold response genes C-REPEAT/DRE BINDING FACTOR 1 ( CBF1 ) and CBF3 (ref. 59 ), and many genes involved in stress and stimulus response are implicated as target genes of JMJ30 and JMJ32 ( Fig. 9b ). It would be interesting to further study the roles of JMJ30 , JMJ32 and FLC in stress responses. FLC is also known to mediate the temperature compensation mechanism of the circadian clock at elevated temperatures by lengthening the circadian period, possibly through regulating the expression of an MYB transcription factor LUX ARRHYTHMO ( LUX ) [60] . During circadian oscillation, the transcriptional feedback loop between the central clock genes CIRCADIAN CLOCK ASSOCIATED 1 ( CCA1 ), LATE ELONGATED HYPOCOTYL ( LHY ) and TIMING OF CAB EXPRESSION 1 ( TOC1 ) forms the core oscillator [61] . Two core clock genes, CCA1 and LHY , directly bind and repress JMJ30 (ref. 41 ), whereas JMJ30, in turn, promotes the expression of the morning-phased clock genes, CCA1 and LHY [42] , forming a negative feedback loop similar to the central CCA1 / LHY / TOC1 oscillation. Taken together, the interactions between FLC , JMJ30 and the circadian clock genes provide a platform for crosstalk between the flowering pathway and circadian regulation to modulate plant responses to fluctuating temperatures. One of the key players in the thermosensory pathway, the repressive H2A.Z occupancy controlling the accessibility of PIF4 , mediates thermosensory responses by wrapping DNA more tightly at lower temperatures, thus negatively affecting PIF4 -mediated transcription [8] , [9] . Although the heat-induced upregulation outcome of the H2A.Z-mediated mechanism fits the FLC expression profile, FLC does not seem to be a PIF4-regulated target gene [62] . On the other hand, recent publications showed that SVP, FLC and different splice variants of FLM form MADS-box heterocomplexes to control flowering time in response to ambient temperature changes [12] , [13] , [14] . The SVP-FLM-β complex delays flowering through the transcriptional repression of FT and SOC1 at low temperatures, which is alleviated by the FLM -δ dominant-negative form at increased temperatures [13] , [14] . SVP may also form a complex with FLC to repress flowering at elevated temperatures, although this is less likely because SVP is rapidly degraded at elevated temperatures [13] . Taken together, our work suggests that JMJ30- and JMJ32-regulated FLC expression, in parallel with temperature-responsive H2A.Z nucleosome occupancy [9] and SVP-FLM cold-sensing pathways [13] , [14] , may function to balance and coordinate flowering time in response to fluctuating temperatures. A recent study showed that flowering in chrysanthemum is repressed at elevated temperatures through the downregulation of one of its floral inducers, FLOWERING LOCUS T-like 3 ( FTL3 ) [63] . Together with our results, this finding suggests that the need for a thermosensory balancing mechanism that represses flowering at elevated temperatures may be conserved, although the molecules involved in the process may differ. When plants are grown in an environment with fluctuating temperatures, the interplay between floral inductive and repressive signals plays a key role in determining the optimal flowering time for reproductive success. All in all, this study provides insights into the regulation of flowering time through FLC heat-inductive expression, which is partly achieved through the activity of H3K27 demethylases, JMJ30 and JMJ32. Plant materials and growth conditions All Arabidopsis thaliana plants used were in the background of the ecotype Columbia (Col). The jmj32-1 (SALK_003313) allele was isolated from the SALK collections from ABRC. The alleles of jmj30-1 (SAIL_811_H12) [41] , [42] , jmj30-2 (GK-454C10) [41] , [42] and flc-3 [36] were described previously. Plants were grown in LDs (16-h light/8-h dark) or SDs (8-h light/16-h dark) at 22 °C or 29 °C. Genotyping primer sequences are shown in Supplementary Table 1 . Total primary rosette leaves before bolting were counted to measure flowering time. Statistical analysis was performed using two-tailed Student’s t -test. Plasmid construction and plant transformation To construct the 35S::JMJ30-HA plasmid, the full-length JMJ30 coding sequence was amplified by primer set XhoI-JMJ30_F and Bsp120I-JMJ30_R ( Supplementary Table 2 ) and cloned into vectors pGREEN-35S-HA [64] using Xho I and Bsp 120I restriction enzymes. Mutagenesis using the primers JMJ30-H326A-F and JMJ30-H326A-R produced the 35S::JMJ30H326A-HA plasmid. The 35S::JMJ32-HA plasmid was constructed similarly, using primer set XhoI-JMJ32_F and Bsp120I-JMJ32_R ( Supplementary Table 2 ), and 35S::JMJ32H174A-HA was constructed through mutagenesis using primers JMJ32-H174A-F and JMJ32-H174A-R. For the pJMJ30::JMJ30-GUS and pJMJ30::JMJ30-HA plasmids, a 6.1-kb JMJ30 genomic fragment (from −2,313 to +3,798; A of the start codon was set as +1) was cloned into pCR8 TOPO vector (Invitrogen) using primers JMJ30-FL_F and JMJ30-FL_R. An Sfo I restriction site was introduced in front of the JMJ30 stop codon through mutagenesis using primers JMJ30-mut_F and JMJ30-mut_R ( Supplementary Table 2 ). GUS or HA fragments were then inserted into the Sfo I site of the pCR8-JMJ30 plasmid. Finally, pJMJ30::JMJ30-GUS and pJMJ30::JMJ30-HA in pCR8 were recombined into pEarleyGate303 and pHGW, respectively, using LR Clonase II (Invitrogen). pJMJ32::JMJ32-GUS plasmid was constructed similarly to pJMJ30::JMJ30-GUS , differing only in that the 5.3-kb JMJ32 genomic fragment (from −3,215 to +2,084) was cloned using primer set JMJ32-FL_F and JMJ32-FL_R, and mutagenesis was performed using primers JMJ32-mut_F and JMJ32-mut_R ( Supplementary Table 2 ). Transgenic plants were generated by floral dipping with Agrobacterium tumefaciens (strain C58C1; with additional pSOUP helper plasmid for transformation of pGREEN-35S::JMJ30-HA ) [65] . RNA extraction and expression analysis For the tissue expression analysis of JMJ30 and JMJ32 , total RNA was isolated from young seedlings, rosette leaves, cauline leaves, stems and inflorescences. For the time-course flowering time gene expression analysis, samples were harvested from aerial parts of 5 DAG to 13 DAG seedlings for WT, jmj30 , jmj32 and jmj30 jmj32 , and 1- to 3-week old seedlings for FRI and FRI jmj30 jmj32 (collected at the end of the light photoperiod). Total RNA was extracted using the RNeasy plant mini kit (Qiagen) according to the manufacturer’s instructions. 2 μg total RNA was used for reverse transcription using the Superscript III RT–PCR system (Invitrogen). RT–PCR with gene-specific primers ( Supplementary Table 3 ) was performed using HotStarTaq DNA Polymerase (Qiagen) on a Thermocycler (Bio-Rad) for 15–25 cycles. Real-time quantitative PCR (qPCR) was performed on an ABI PRISM 7900HT sequence detection system (Applied Biosystems) using the KAPA SYBR FAST ABI Prism qPCR Master Mix (KAPA Biosystems). Tip41-like (AT4G34270) was used as an internal reference gene [66] . The relative expression of a gene of interest is calculated as 2 −ΔΔCT [ΔΔ C T =Δ C T (experimental sample)−Δ C T (control sample); Δ C T = C T (gene of interest)– C T ( Tip41-like )]. Statistical analysis was performed using two-tailed Student’s t -test. The primer sequences are shown in Supplementary Table 3 . GUS staining GUS staining was performed as previously described with slight modifications [67] . Briefly, plant tissues were fixed by incubating in ice-cold 90% acetone for 30 min and rinsed with rinsing solution (50 mM NaPO 4 , pH 7.2, 0.5 mM K 3 Fe(CN) 6 and 0.5 mM K 4 Fe(CN) 6 ). The tissues were then stained in staining solution (50 mM NaPO 4 , pH 7.2, 0.5 mM K 3 Fe(CN) 6 , 0.5 mM K 4 Fe(CN) 6 , 2 mM X-gluc) at 37 °C overnight. After staining, the tissues were placed in fixation solution (50% ethanol, 5% acetic acid and 3.7% formaldehyde) at room temperature overnight and transferred to 100% ethanol the following day. For histological analysis, the tissues were mounted on slides with clearing solution (Hoyer’s solution containing 30 ml water, 100 g chloral hydrate, 7.5 g gum Arabic, 5 ml glycerol) and observed under a SteREO Discovery.V12 Stereomicroscope (Zeiss) with images taken with an AxioCam ICc 3 (Zeiss). ChIP assays ChIP experiments were performed as previously described with minor modifications [67] , [68] . Briefly, total chromatin was extracted from 8 DAG seedlings (collected at the end of the light photoperiod) and immunoprecipitated using anti-HA (Santa Cruz Biotechnology, #sc-7392) and normal mouse IgG as a control (Santa Cruz Biotechnology, #sc-2025), or anti-H3K27me3 (Millipore, #07-449) and anti-H3 as a control (Abcam, #ab1791). Antibody dilutions of 1:200 were used (5 μl antibody in 1 ml of immunoprecipitation reaction). DNA fragments were recovered by phenol–chloroform extraction. qPCR with gene-specific primers ( Supplementary Table 3 ) was performed on an ABI PRISM 7900HT sequence detection system (Applied Biosystems) using the KAPA SYBR FAST ABI Prism qPCR Master Mix (KAPA Biosystems). The results were first normalized to an internal control Mutator-like transposon (AT4G03870). For the histone modification ChIP, the relative enrichment was calculated by taking the ratio of DNA immunoprecipitated with anti-H3K27me3 antibody with that of anti-H3 antibody. Similarly, the ChIP relative enrichment of JMJ30-HA binding was calculated from the ratio between anti-HA antibody and normal mouse IgG immunoprecipitated DNA. Statistical analysis was performed using two-tailed Student’s t -test. Immunolocalization The isolation of nuclei and in situ immunolocalization of chromatin proteins were performed as described with minor modifications [69] . Young leaves from pJMJ30::JMJ30-HA transgenic plants were fixed in ice-cold 4% formaldehyde Tris buffer for 20 min, rinsed and chopped into a fine suspension in LB01 buffer (15 mM Tris–HCl, pH 7.5, 2 mM EDTA, 0.5 mM spermine, 80 mM KCl, 20 mM NaCl, 0.1% Triton X-100). The sample suspension was air-dried on glass slides. Each slide was blocked with 1% BSA in 1 × PBS before incubating with mouse anti-HA antibody (Santa Cruz Biotechnology, #sc-7392) and later with CF555 goat anti-mouse IgG antibody (Biotium, #20030). A dilution of 1:200 is used for both primary and secondary antibodies. The slides were stained with DAPI and imaged with a Leica TCS SP5 confocal microscope (Leica). Immunolocalization of protoplasts were performed as described [70] . Mouse anti-HA (Santa Cruz Biotechnology, #sc-7392) and rabbit anti-H3K27me3 (Millipore, #07-449) antibodies were used as primary antibodies, whereas CF555 goat anti-mouse IgG (Biotium, #20030) and CF488 goat anti-rabbit IgG antibodies (Biotium, #20012) were used as secondary antibodies. A dilution of 1:200 is used for both primary and secondary antibodies. The slides were stained with DAPI and imaged with a Leica TCS SPE confocal microscope (Leica). In vitro histone demethylase assays Recombinant JMJ30-HA was transiently overexpressed in tobacco leaves and immunoaffinity-purified using anti-HA beads (Sigma, A2095). Histone demethylase assay was performed as previously described [25] , [29] . Briefly, the purified JMJ30-HA enzymes and substrate calf thymus histone (4 μg) were co-incubated in a 20-μl reaction mix (20 mM Tris–HCl, pH 7.5, 150 mM NaCl, 50 μM Fe(NH 4 ) 2 (SO 4 ) 2 , 1 mM α-KG, 2 mM ascorbate) for 4 h at 37 °C. The reaction products were analysed by western blotting using the following antibodies: anti-H3K27me3 (Millipore, #07-449), anti-H3K27me2 (Millipore, #07-452), anti-H3K27me1 (Millipore, #07-448), anti-H3K9me3 (Millipore, #07-442), anti-H3K9me2 (Millipore, #07-441), anti-H3K4me3 (Millipore, #07-473), anti-H3K4me2 (Millipore, #07-030), anti-H3K36me3 (Abcam, #ab9050), anti-H3K36me2 (Abcam, #ab9049) and anti-H3 (Abcam, #ab1791). A dilution of 1:1,000 is used for primary antibodies and 1:10,000 for secondary antibodies. Band intensity was calculated using ImageJ. Uncropped scans of western blot results are shown in Supplementary Fig. 13 . In vivo histone demethylase assays The protoplast transformation and in vivo histone demethylase assays were conducted as previously described [70] . Briefly, JMJ30-HA, JMJ30H326A, JMJ32-HA and JMJ32H174A were transiently overexpressed in Arabidopsis leaf protoplasts through polyethylene glycol (PEG)-mediated transformation. After one day, nuclei were isolated from the protoplasts and air-dried on the slide. Immunostaining was performed as described [69] by incubating each slide with mouse anti-HA (Santa Cruz Biotechnology, #sc-7392) and rabbit anti-H3K27me3 (Millipore, #07-449) antibodies, and then with CF555 goat anti-mouse IgG (Biotium, #20030) and CF488 goat anti-rabbit IgG antibodies (Biotium, #20012). A dilution of 1:200 is used for both primary and secondary antibodies. The slides were stained with DAPI and imaged with a Leica TCS SP8 confocal microscope (Leica). The intensities of at least 50 pairs of closely located JMJ-HA-transformed and non-transformed nuclei were analysed using ImageJ. Data were presented as a relative intensity of transformed/non-transformed nuclei and statistical analysis was performed using two-tailed Student’s t -test. Protein expression assays Samples for the time-course JMJ30-HA protein expression experiment were harvested from aerial parts of 9 DAG pJMJ30::JMJ30-HA or 35S::JMJ30-HA seedlings. The JMJ30-HA protein stability assay with CHX and MG132 was performed as described [13] . Total protein was extracted by grinding plant tissues in liquid nitrogen and resuspending in an equal volume of 2 × SDS loading buffer (4% SDS, 20% glycerol, 0.125 M Tris pH 6.8, 0.2% bromophenol blue, 200 mM β-mercaptoethanol). Protein samples were incubated at 95 °C for 10 min and then centrifuged for 10 min at 12,000 g . The supernatant was used for western blots using anti-HA-HRP (Santa Cruz Biotechnology, #sc-7392 HRP) using a dilution of 1:2,000. Band intensity was calculated using ImageJ. Uncropped scans of western blot results are shown in Supplementary Fig. 13 . Microarray analysis For genome-wide expression analysis, two replicates of WT, jmj30-2 jmj32-1 and 35S::JMJ30-HA samples were analysed by NimbleGen 12 × 135K arrays (Roche). Total RNA was extracted from aerial parts of 13 DAG seedlings with the RNeasy plant mini kit (Qiagen), and double-stranded cDNA was synthesized using the SuperScript double-stranded cDNA synthesis kit (Invitrogen). cDNA samples were Cy3-labelled and hybridized following the manufacturer’s instructions (Roche Nimblegen). Gene expression was analysed by Arraystar (DNAStar), and genes showing at least a 1.5-fold change within a 90% confidence interval were considered to be differentially expressed and were presented in Supplementary Data 1 and Supplementary Data 2 . Gene enrichments with H3K27me3 target were tested with Fisher’s exact test using R. Dot blot The specificity of the anti-histone antibodies was tested by dot blot ( Supplementary Fig. 12 ). Different amount of biotin-labelled histone peptide are blotted onto a nitrocellulose membrane. Western blot analyses were then performed using the anti-histone antibodies: anti-H3K27me3 (Millipore, #07-449), anti-H3K4me3 (Millipore, #07-473) and anti-H3K36me3 (Abcam, #ab9050). A dilution of 1:1,000 is used for primary antibodies and 1:10,000 for secondary antibodies. The control experiment was probed using Strepavidin-HRP (Thermo Scientific Pierce, #21130) using a dilution of 1:1,000. The histone peptide used include: Biotinylated Histone H3 Peptide residues 1−21 (Epigentek, #R−1004−100), Biotinylated Histone H3 Peptide residues 21−44 (Epigentek, #R−1006−100), Biotinylated Trimethyl Histone H3K4 Peptide (Epigentek, #R−1023−100), Biotinylated Trimethyl Histone H3K9 Peptide (Epigentek, #R−1029−100), Biotinylated Trimethyl Histone H3K27 Peptide (Epigentek, #R−1035−100) and Biotinylated Trimethyl Histone H3K36 Peptide (Epigentek, #R−1050−100). How to cite this article: Gan, E.-S. et al . Jumonji demethylases moderate precocious flowering at elevated temperature via regulation of FLC in Arabidopsis . Nat. Commun. 5:5098 doi: 10.1038/ncomms6098 (2014). Accession codes: The NimbleGen 12 × 135 K expression array data sets are deposited in the NCBI Gene Expression Omnibus (GEO) under the accession code GSE51898 .